Recurrentde novomutations implicate novel genes underlying simplex autism risk Autism spectrum disorder (ASD) has a strong but complex genetic component. Here we report on the resequencing of 64 candidate neurodevelopmental disorder risk genes in 5,979 individuals: 3,486 probands and 2,493 unaffected siblings. We find a strong burden of de novo point mutations for these genes and specifically implicate nine genes. These include CHD2 and SYNGAP1 , genes previously reported in related disorders, and novel genes TRIP12 and PAX5 . We also show that mutation carriers generally have lower IQs and enrichment for seizures. These data begin to distinguish genetically distinct subtypes of autism important for aetiological classification and future therapeutics. Over the past several years, we and others have used whole-exome sequencing of families with a single autism spectrum disorder (ASD) proband to identify de novo coding mutations [1] , [2] , [3] , [4] , [5] , yielding hundreds of new candidate ASD risk genes. However, recurrent disruptions have only been observed in a handful of genes. Furthermore, cohort sizes are approaching a scale where even recurrence is not necessarily significant when sequencing the entire exome. We previously demonstrated using modified molecular inversion probes (MIPs) that we could economically resequence a modest number of candidate genes across large cohorts [6] . We concurrently developed a statistical approach to rigorously implicate ASD risk genes based on a recurrent disruption model that takes into account known and predicted mutational biases and multiple hypothesis testing. Here we further explore this paradigm by successfully resequencing 64 genes in 4,260 new and 1,719 previously exome-sequenced individuals from two large family-based simplex ASD cohorts. We compare de novo mutation burden between probands and unaffected siblings, finding a strong enrichment for new mutations overall, especially those that are predicted to be more severe. Probands with mutations have a lower intelligence quotient (IQ) distribution and are enriched for reports of seizures. Based on our recurrent disruption model, we specifically implicate nine individual genes with ASD risk. We believe that firmly implicating new genes that are mutated in a sizable fraction of children with ASD provides the motivation for further functional and translational studies of these specific genes. Resequencing of 64 genes in large simplex ASD cohorts We selected candidate genes from previously published reports and our own unpublished data (discovery set). These included de novo mutation calls from exome sequencing of 1,308 probands (1,157 ASD (208 from (ref. 7 )) and 151 intellectual disability (ID)) and 803 unaffected siblings or controls (195 from (ref. 7 )) [1] , [2] , [3] , [4] , [5] , [6] , [8] , [9] . We selected genes that were recurrently disrupted or with at least one putative severe (nonsense, canonical splice site or small insertion/deletion (indel)) event found exclusively in probands. We excluded genes based on high-predicted mutability or known associations with likely unrelated conditions in Online Mendelian Inheritance in Man (OMIM). We ranked genes based on recurrence, presence in protein–protein interaction (PPI) networks, predicted role in chromatin regulation and our previously unpublished exome data (see Methods section). 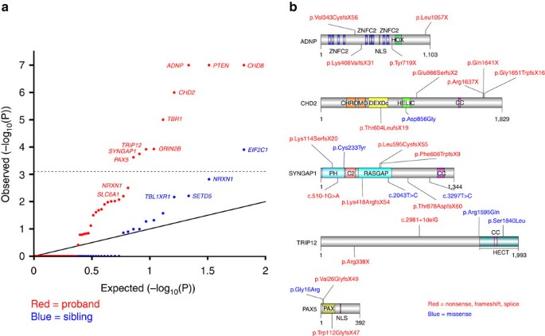Figure 1: smMIP resequencing of 64 genes implicates specific genes in ASD. (a) Quantile–quantile plot comparing the individual gene recurrence mutation simulation results from the MIP-only samples (2,757 ASD probands and 1,733 unaffected siblings) to a uniform distribution (see Methods section). Proband data are plotted in red and sibling data in blue. Proband data implicate nine genes as significantly disrupted in ASD. Dashed line indicates a Holm–Bonferroni corrected significance level. (b) Protein diagrams of five genes with significant recurrentde novomutations. Annotated protein domains are shown (coloured blocks) for the largest protein isoforms. Mutations shown above the protein structure were newly identified in this study using MIPs. Mutations shown below the protein structure have been previously reported from exome sequencing of ASD/ID cohorts or MIP-based resequencing6. Red variants are nonsense, frameshifting or splice site. Domains: ZNFC2, zinc finger; NLS, nuclear localization signal; HOX, homeodomain; CHROMO, chromatin organization modifier; DEXDc, DEAD-like helicases superfamily; HELIC, helicase superfamily C-terminal; CC, coiled coil; PH, pleckstrin homology; RASGAP, GTPase-activator for Ras-like GTPases; HECT, homologous to E6-AP carboxyl terminus; PAX, paired box. The final set consisted of 64 candidate genes ( Supplementary Table 1 )—56 novel neurodevelopmental candidates and 8 genes screened previously in a subset of the samples [6] . We designed MIPs using an improved design implementation [10] and also incorporated molecular tagging [11] . Specifically, the MIP backbone contains a degenerate region, such that each independent MIP capture event is associated with a single-molecular (sm) tag that can be used to identify PCR duplicates and to more accurately count mutation allele frequencies—analogous to PCR subcloning. The final design included 2,928 smMIPs that were individually synthesized, pooled and tested using control DNA. Probe concentrations were modified based on empirical performance to generate a rebalanced working probe set. We targeted two well-described simplex (sporadic) ASD cohorts that meet ASD criteria on both of the current gold-standard autism diagnostic assessments (Autism Diagnostic Interview-Revised (ADI-R) and Autism Diagnostic Observation Schedule (ADOS)), the Simons Simplex Collection (SSC) [12] and The Autism Simplex Collection (TASC) [13] . Exome sequencing was available for a portion of the SSC individuals, which was used as the discovery set ( Supplementary Table 2 ). While 8 of the 64 targeted genes overlap our previous study [6] , here we captured and sequenced ~2,600 individuals that had not been previously MIP or exome-sequenced, including all of TASC ( n =921 probands and n =124 siblings), unaffected siblings from the SSC ( n =1,638) and a small number of additional SSC probands. In addition, to identify de novo mutations that may have been missed by exome sequencing, we resequenced 974 ASD probands and 773 unaffected siblings from this exome discovery set using our smMIP pool. In total, 3,486 probands (2,527 MIP sequenced and 959 MIP and exome-sequenced) and 2,493 siblings (1,733 MIP sequenced; 760 MIP and exome-sequenced) passed capture and other QC measures ( Supplementary Table 2 ; see Methods section). We discovered >1,400 rare variants predicted to alter protein sequence or gene splicing and evaluated these sites in relevant parents by resequencing with smMIP subpools or the full probe set. Potential de novo events were confirmed using Sanger sequencing and paternity was firmly established using common variant calls across the full probe set. Mutation analysis in the MIP-only ASD data set For our primary analysis of mutation burden and individual gene recurrence, we restricted our analysis to only the newly sequenced 2,527 probands and 1,733 siblings. In probands, we discovered 56 de novo mutations in 27 of the 64 candidate genes ( Table 1 and Supplementary Data 1 ). This total includes 16 mutations in the eight genes screened previously in a subset of the samples [6] . The most mutated gene was CHD8 with 11 total mutations (20% of all proband de novo mutations). In addition, we observed three or more mutations in PTEN , TBR1 , SYNGAP1 , CHD2 , ADNP , GRIN2B and TRIP12 . In stark contrast, we observed only 14 de novo mutations in unaffected siblings for 11 of the 64 genes. No genes were found to have >2 de novo events in siblings. Importantly, the increased sensitivity of the smMIPs allowed for identification of five events (three in probands and two in siblings) with skewed allele frequencies likely reflecting mosaic mutations ( Supplementary Data 1 ). Most notable was a heterozygous nonsense mutation in ADNP identified in a proband that shows evidence of low-level mosaicism (~10% allele frequency) in the child’s mother ( Supplementary Fig. 1 ). Table 1 Summary of proband de novo mutations for exome and MIP sequencing results for individual genes that were significantly deviated from the simulation-based expectation. Full size table The overall rate of protein-altering mutations for these 64 genes is 2.7-fold greater in the probands compared with the unaffected siblings ( Supplementary Table 3 ; 0.022 versus 0.0081 mutations per individual; rate ratio test, one-sided P value=0.000199; 1.4% differential). The distribution of proband mutations is markedly skewed towards mutations predicted to be severe (nonsense, splice site and indels) relative to missense changes (observed 46.4% severe; expected 16% severe; binomial P( X ≥26)=9.1 × 10 −8 ), while the sibling mutations fit the null expectation (observed 14.3% severe). Consistent with this, the rate of severe mutations is more markedly skewed in probands compared with unaffected siblings (0.010 versus 0.0012 mutations per individual; 8.92-fold; 95% confidence interval (CI) 2.61-Inf; rate ratio test, one-sided P value=8.8 × 10 −5 ), while the rate of missense mutations is only modestly greater (0.012 versus 0.0069 mutations per individual; 1.71-fold; 95% CI 0.94-Inf; rate ratio test, one-sided P value=0.07285). We also evaluated the observed results in the context of a recurrent mutation simulation model that takes into account mutation type (missense versus severe) and differences in relative mutation rates between genes [6] . Importantly, this model can provide relative confidence estimates for each gene based on the current evidence. Others have proposed similar models and approaches [14] , [15] , [16] . Again, we observed a marked mutation burden in probands, as simulation reported on average only 6.6 missense mutations (versus 30 observed) and 0.82 severe mutations (versus 26 observed; Supplementary Table 4 ). When evaluating the individual genes, nine were significantly mutated in the probands, implicating these loci in ASD risk to various degrees ( Fig. 1 and Supplementary Fig. 2 ). We previously reported four of these genes— CHD8 , PTEN , TBR1 , GRIN2B— as significant in a smaller ASD cohort, and one additional gene, ADNP , was previously insignificant [6] . The other significant genes include CHD2 and SYNGAP1 , previously reported in related disorders with potential ASD phenotypic overlap [14] , [16] , [17] , [18] , [19] , [20] , and novel genes TRIP12 and PAX5 ( Fig. 1b ). In contrast, in the sibling analysis, only one gene, EIF2C1 , was marginally significant ( Fig. 1a ). Figure 1: smMIP resequencing of 64 genes implicates specific genes in ASD. ( a ) Quantile–quantile plot comparing the individual gene recurrence mutation simulation results from the MIP-only samples (2,757 ASD probands and 1,733 unaffected siblings) to a uniform distribution (see Methods section). Proband data are plotted in red and sibling data in blue. Proband data implicate nine genes as significantly disrupted in ASD. Dashed line indicates a Holm–Bonferroni corrected significance level. ( b ) Protein diagrams of five genes with significant recurrent de novo mutations. Annotated protein domains are shown (coloured blocks) for the largest protein isoforms. Mutations shown above the protein structure were newly identified in this study using MIPs. Mutations shown below the protein structure have been previously reported from exome sequencing of ASD/ID cohorts or MIP-based resequencing [6] . Red variants are nonsense, frameshifting or splice site. Domains: ZNFC2, zinc finger; NLS, nuclear localization signal; HOX, homeodomain; CHROMO, chromatin organization modifier; DEXDc, DEAD-like helicases superfamily; HELIC, helicase superfamily C-terminal; CC, coiled coil; PH, pleckstrin homology; RASGAP, GTPase-activator for Ras-like GTPases; HECT, homologous to E6-AP carboxyl terminus; PAX, paired box. Full size image Mutation analysis in combined ASD data sets As a secondary analysis, we evaluated the full data set of ASD exome plus MIP-identified events. Overall smMIPs showed good sensitivity, detecting 54/58 de novo events previously identified and 10 new de novo mutations not previously identified in these individuals by exome sequencing. The smMIP false negatives were the result of low coverage or poor quality data for these specific sites. The severe mutation rate is ~28-fold higher in probands ( Supplementary Table 3 ; probands: 0.022, siblings: 0.00079 and differential: 2.1%), and missense mutations are ~2-fold in excess (probands: 0.0136, siblings: 0.0060 and differential: 0.76%). Overall, the combined differential of both mutation types is ~3%, although this is likely an overestimate as it is inclusive of nominating events in all genes. In the proband simulation, eight genes with recurrent mutations reach a conservative Bonferroni genome-wide significant threshold, including DYRK1A [6] ( Supplementary Fig. 3 and Supplementary Table 5 ). Despite not reaching significance in the resequencing data alone, DSCAM has three severe de novo mutations ( Supplementary Fig. 4 ). If eventually implicated further, DSCAM would join DYRK1A as genes in the Down’s syndrome critical region [21] , [22] that are also risk factors for ASD, suggesting a dosage reciprocity effect for these two critical genes—where increases in copy number associate with Down’s syndrome/ID and reductions associate with ASD. Common mutation comorbidities The association of lower IQ with more severe de novo mutations en masse has been described repeatedly [1] , [23] , [24] . We discover similar skewed (from the Gaussian distribution) mean and median IQ distributions for the non-mutation carriers in both SSC and TASC cohorts (SSC: 85.6/89 and TASC: 84.6/86). We find the IQ distribution of the mutation carriers ( n =52) to be significantly lower compared with the mutation-negative samples, with approximately half in the ID range (mean/median: 69.2/72, Wilcox P <1 × 10 −4 ; Supplementary Fig. 5 ). This distribution deviation is true for both missense and severe mutations, which is notable given the weak signal for missense mutations and lower IQ exome-wide. Among the nine significant genes from the primary analysis, only three have mutation carriers exclusively in the ID IQ range: ADNP (range 19–55), GRIN2B (range 55–65) and TRIP12 (range 53–72). Based on the strict autism inclusion criteria (ADI-R+ADOS), we can be confident that these cases meet the current clinical criteria for ASD. How generalizable these genetic risk factors will be to individuals with ID or developmental delay that do not meet autistic diagnostic criteria is an important area of future research that will require targeted sequencing of large cohorts of patients with developmental delay [25] . Seizures are a comorbid condition often associated with ASD [26] . In the primary data (MIP-only) 98/2,282 (4.3%) probands without mutations (with reports) have a history of seizures or have a parent report of possible seizures. Among de novo mutation carriers, 6/51 (11.8%) are positive for seizures, which is a significant enrichment (Fisher’s exact test, P =0.024, odds ratio: 2.971, 95% CI: 1.112–7.481). In the full data set (including the exome data samples, which may include some selection bias) for those with available seizure history data, a stronger association is seen. Seizures are reported at a much higher rate in the mutation carriers (23/123 (18.7%)) versus those without mutations (151/3611 (4.2%); Fisher’s exact test, P <0.00001, odds ratio: 5.2, 95% CI: 3.3–8.5). Moving from candidate gene discovery to gene validation has been a major challenge for neurodevelopmental/psychiatric genetics. With sets of high-confidence risk genes and the ability to recontact and evaluate individual patients, it is now feasible to use this type of genotype-first approach to link significant genotypes to clinical phenotypes in ASD and related disorders [27] . Moreover, specific genotypes may span our current diagnostic categories in unexpected ways. Initial efforts in this vein with relatively small cohorts (<10) have already proven fruitful. Through a parallel study, we showed that CHD8 , a chromatin remodelling factor, is linked to a clinical phenotype, including significant macrocephaly, distinct facial features and gastrointestinal defects, which can be modelled in zebrafish [28] . In this study, we identified seven novel CHD8 mutations, some presenting with phenotypes similar to those previously reported ( Supplementary Data 2 ). However, we also identified missense mutations (not previously observed), 3/4 of which do not demonstrate reported macrocephaly. Similarly, mutations in ADNP , a transcription factor involved in the SWItch/Sucrose NonFermentable (SWI/SNF) remodelling complex, are linked to a shared clinical phenotype including ID and a characteristic facial dysmorphism [29] . In our case, the four probands with ADNP mutations all have a confirmed ASD diagnosis and are also severely impaired cognitively ( Supplementary Data 2 ). Two genes reported here, CHD2 and SYNGAP1 , have been implicated now across several neurodevelopmental disorders. SYNGAP1 de novo mutations have been observed in patients with ID, with or without autism and/or seizures, and epileptic encephalopathies, again with or without ASD features [17] , [18] , [19] . CHD2 , chromodomain helicase DNA binding protein 2, is a chromatin remodelling factor for which de novo deletions have been associated with recurrent clinical symptoms, including developmental delay, ID, epilepsy, behavioral problems and ASD-like features without characteristic facial gestalt or brain malformations [14] , [20] , and de novo point mutations have been associated again in epileptic encephalopathies with ID and occasionally ASD [17] . In our four CHD2 mutation carriers, all have confirmed autism that is skewed towards higher ASD severity, according to the clinician-derived ADOS-calibrated severity scores, as well as parent and teacher reporting on the Social Responsiveness Scale, three have reports of seizures, and there are a range of cognitive impairments. In contrast, of the four SYNGAP1 mutation carriers none report seizures (one unknown). Interestingly, similar methods have now firmly implicated SYNGAP1 in both ID [16] and ASD (presented here) based on independent data sets/analyses. These efforts have also contributed novel candidates for clinical follow-up, including the genes TRIP12 and PAX5 . Very little is known about what role TRIP12 , thyroid hormone receptor interactor 12, may play in neurodevelopment having been primarily described as a protein with E3 ubiquitin–protein ligase activity involved in the ubiquitin fusion degradation pathway and the regulation of DNA repair [30] . PAX5 , paired box protein 5, is a transcription factor and has been shown as significantly downregulated in bipolar disorder postmortem hippocampal extracts [31] . Conditional knockout of Pax5 in GABAergic neurons in mice highlight the necessity for this gene in normal ventricular development [32] , further promoting a specific role for Pax5 in the aetiology of ASD. Preliminary analysis based on existing data shows that TRIP12 mutation carriers all have ASD and ID ranging from mild-to-moderate severity, while the individuals with PAX5 demonstrate a higher range of cognitive ability from borderline to average intelligence concomitant with ASD. Individuals with both genes display variation in physical features (for example, head size), presence of regression, language ability and other psychiatric features. While this study focused on autism cohorts, we note that combining our results with other comorbid phenotypes, such as ID, reveals additional genes such as PPP2R5D . In addition to autism, the preliminary data on both individuals with PPP2R5D highlight short stature and problems with excessive sleepiness, warranting further follow-up. The ongoing genetic classification of distinct subtypes of neurodevelopmental disorders promises to revolutionize not only our understanding of the biological nature of these conditions and their expressivity but also the precision treatment of patients moving forward. Human subjects All participants completed informed consent/assent before participation in the original data collection study [12] , [13] . Approval for sequencing was obtained from each local institutional review board. All samples and phenotypic data were de-identified before release. DNA samples were obtained from the Rutgers University Cell and DNA Repository through the Simons Foundation Autism Research Initiative (SSC) or National Institute of Mental Health (TASC). The human subjects in this project were deemed exempt from IRB approval by the University of Washington Human Subjects Division. Families in the MIP-only category were excluded from the study if the proband did not meet criteria for ASD on ADI-R and ADOS, if multiple possibly affected individuals were indicated, and/or if both parents were not available. We did not exclude any individuals from the previously published exome data sets. Gene selection We combined and harmonized annotations of de novo mutation calls from exome sequencing of 1,308 probands (1,157 ASD (208 from (ref. 7 )), and 151 ID) and 803 unaffected siblings or controls (195 from (ref. 7 )) [1] , [2] , [3] , [4] , [5] , [8] , [9] . We further annotated the 954 genes with at least one predicted protein-altering mutation in probands with mutability estimates and known disease/disorder associations. Similar to reported previously, we conducted a PPI analysis using either the set of genes as nodes with either (1) one proband truncating or splice-disrupting event (trunc network), or (2) missense (Grantham score ≥50 and Genomic Evolutionary Rate Profiling (GERP) score ≥3 or Grantham score ≥85), other indels, and truncating events (severe network). Human PPI data were collected from GeneMANIA [33] on 29 August 2011. Only direct physical interactions from the Homo sapiens database were considered. We then selected 64 genes prioritizing those that were recurrently disrupted or with at least one putative severe (non-missense) event found exclusively in probands, low predicted mutability, membership in the major connected component of either PPI analysis set, predicted role in chromatin regulation, or novelty (that is, for our own unpublished exome data; Supplementary Tables 6 and 7 , and Supplementary Figs 6 and 7 ). We excluded a small number of strong candidates being screened by other studies. For example, SCN2A , POGZ and KATNAL2 were all identified with multiple mutations in the discovery set. We elected not to include these in our set because we were aware on an ongoing effort by others to sequence these genes. The final set included eight genes screened previously in a subset of the samples [6] . MIP design and testing All smMIPs were designed with an updated scoring algorithm described recently [10] . MIP arms+predicted gap fill were set to total a fixed length of 162 base pairs (bp). Individual arms ranged from 15 to 30 bp. Oligonucleotides (IDT, Coralville, IA) were ordered with five degenerate bases between the end of the common linker and the extension arm allowing for a maximum theoretical non-duplicate coverage of (4 5 =1,024). Probes were pooled by gene and then combined in equal molar ratios and phosphorylated (1 × pool). After initial testing, the bottom 400 performing probes were repooled and phosphorylated (50 × pool). The next 242 poorest performing probes were repooled and phosphorylated (10 × pool). A final working probe pool was then generated by combining the three pools so that the final concentration of each MIP in the 10 × and 50 × initial pools was a 10- or 50-fold excess relative to the 1 × pool concentration. Multiplex capture and amplification of targeted sequences Hybridization of smMIPs to genomic DNA, gap filling and ligation were performed in one 25 μl reaction of 1 × Ampligase buffer (Epicentre, Madison, WI) with 120 ng of genomic DNA, 0.32 μM dNTPs, 0.5 × of Hemo KlenTaq (0.32 μl; New England Biolabs, Inc., Ipswich, MA), one unit of Ampligase (Epicentre) and MIPs. MIP concentration was based on a ratio of 667 copies of each MIP to each haploid genome copy, based on the 1 × pool concentration. Reactions were incubated at 95 °C for 10 min then at 60 °C for 18 h. Exonuclease treatment and amplification of the captured DNA was performed as previously described [6] . We pooled 5 μl of ~96 different bar coded libraries together and purified the pools with 0.8 × AMPure XP beads (Beckman Coulter, Brea, CA) according to the manufacturer’s protocol. Libraries were resuspended in 100 μl of 1 × EB (Qiagen, Valencia, CA). Pools were quantified in duplicate using the Qubit dsDNA HS Assay (Life Technologies, Grand Island, NY). Multiple libraries were combined to create the final megapools of ~192 individual capture reactions for sequencing. One lane of 101-bp paired-end reads was generated for each megapool on an Illumina HiSeq 2000 according to manufacturer’s instructions. MIP sequencing analysis Sequencing reads were analysed as described previously [6] with minor modifications. The 5-bp degenerated sequence was removed from the beginning of read2 and added to the index bar code to create a sample-tag index. For primary single-nucleotide variation, indel, and target coverage analysis, reads were trimmed to 81 bp before mapping. Indels were also called by mapping the full-length reads. After mapping, read-pairs with incorrect pairs and insert sizes were removed. For capture events with identical tag sequences, only the read-pair with the highest sum of quality scores was used. MIP targeting arm sequences were then removed. On average, >95% of target coding regions had ≥10 × coverage. Coverage distributions were generally consistent across plates/samples ( Supplementary Figs 8–11 ) and between proband and sibling samples when analysed by gene ( Supplementary Figs 12–15 ). Captures with <75% of the target at greater than 10-fold coverage were removed from analysis. Single-nucleotide variation calls required a minimum of eightfold coverage with a consensus or variant quality score of 30 or higher and an allele balance ≤0.80 (considering Q20 bases only). Indel calls required at least 25% of reads to support an event. Variants were removed from the potential de novo validation set if present in Exome Variant Server (ESP6500SI-V2), multiple independent families or siblings from the same family. Validations Rare, potentially protein-altering events (nonsense, splice site, indel and missense) in children were tested for inheritance status by MIP-based resequencing of their parents using subpools of MIPs grouped by gene, containing ~6–13 genes per pool. Parent samples/sites that failed using the subpools were captured using the full probe set. Variants that appeared de novo or failed the full pool capture were further validated with PCR and Sanger sequencing. Samples were removed if non-paternity was suspected or parental DNA was absent or failed to amplify. Statistics Comparisons of de novo rates in probands versus siblings were compared using the exact rate ratio test (one-sided) implemented in the R package rate ratio.test. For recurrence mutation simulation, we used the same probabilistic framework developed previously [6] that incorporates the overall rate of mutation in coding sequences, estimates of relative locus-specific rates based on human–chimpanzee fixed differences in each gene’s coding and splice sequences, and other factors that may influence the distribution of mutation classes, for example, codon structure. We simulated the location of random mutations using this framework based on the number of samples screened and an overall protein-altering mutation rate of 0.9187 events per proband [1] . We then compared our observed (obs) data to the simulation (sim) using counts of two classes of events (1) missense and (2) severe (nonsense, splice site or indel). For gene i , we calculated the probability of observing or more of any protein-altering events, and among them or more severe events, from Z simulations (equation (1)). Accession codes: Raw sequencing data have been deposited in the National Database for Autism Research under the accession code NDARCOL2130. How to cite this article: O'Roak, B. J. et al. Recurrent de novo mutations implicate novel genes underlying simplex autism risk. Nat. Commun. 5:5595 doi: 10.1038/ncomms6595 (2014).